Nematode-derived drosomycin-type antifungal peptides provide evidence for plant-to-ecdysozoan horizontal transfer of a disease resistance gene Drosomycin-type antifungal peptides (DTAFPs) are key innate immunity components of Drosophila and plants and confer resistance to fungal infection. Here we report the discovery of a multigene family of DTAFPs, comprising of 15 members (termed cremycin-1 to crymycin-15), in the fruit nematode Caenorhabditis remanei . Cremycins share highly similar amino-acid sequences and identical precursor organization to drosomycins. Of the 15 cremycin genes, 10 are found to be transcriptionally active and 6 are upregulated after fungal challenge. Synthetic cremycin-5 is active on filamentous fungi and a series of clinical isolates of human pathogenic yeasts and exhibits low haemolysis and high serum stability. The specific distribution of DTAFPs in a clade of moulting animals (Ecdysozoa), including Arthropoda, Nematoda and Tardigrada, together with the widespread presence in plants but the absence in fungi and protozoans, provides evidence for horizontal transfer of a disease resistance gene between plants and ecdysozoans. D rosophila fruitflies larvae are saprophagous insects of rotting fruits where they compete with some saprobiotic filamentous fungi for the same decaying materials [1] . In a long-term antagonistic interaction with fungi, Drosophila have evolved a set of highly efficient immune system to deal with potential fungal infections [2] , in which drosomycin and six additional paralogs (drosomycin-1 to drosomycin-6) constitute a multigene family of core components fighting against a broad spectrum of filamentous fungi [3] , [4] , [5] . The deletion of drosomycin led to a significantly decreased survival rate of Drosophila melanogaster in the presence of fungi, indicating its role in disease resistance [6] . Drosomycins are synthesized as protein precursors that are then processed into mature peptides of 42–46 residues after removal of a signal peptide. Structure-function relationship studies have highlighted eight key amino-acid sites involved in the interaction of drosomycin with fungi [7] . These Drosophila peptides belong to the members of a large γ-thionin (also known as plant defensin) family with structural similarity to invertebrate defensins and scorpion toxins targeting ion channels [3] , [8] . All these peptides adopt a common cysteine-stabilized α-helical and β-sheet (CSαβ) structure characterized by a well-defined two or three-stranded antiparallel β-sheet and a short α-helix with a similar disulphide bridge pattern [9] . Whereas in the animal Kingdom only the melanogaster species group of Drosophila (subgenus Sophophora) was found to contain DTAFPs [10] , in the plant Kingdom DTAFPs exist in nearly all the species [11] . In spite of clear homology and extensive research for nearly 20 years [3] , [4] , [5] , the evolutionary history of DTAFPs in plants and Drosophila remains unsolved. On the basis of the prediction that three hypothetical proteins from fungi have similar structure to plant and Drosophila DTAFPs, we tentatively proposed that all these molecules might originate from a common ancestry [12] , [13] . However, a detailed analysis revealed no detectable sequence similarity between these fungal proteins and DTAFPs [12] . When the fungal sequences were used as queries against the GenBank database with default parameters [14] , no any DTAFPs were returned as hits, and vice versa . These observations provide convincing evidence for their structural analogy other than evolutionary relationship. Alternatively, a patchy distribution (presence or absence patterns) of DTAFPs in plants and Drosophila together with tight association of the fruitflies with plants (i.e., fruits) raises a serious consideration of the possibility of plant-to- Drosophila horizontal gene transfer (HGT, also called lateral gene transfer) [15] . Here we report the discovery and functional characterization of a multigene family of DTAFPs from the fruit nematode Caenorhabditis remanei [16] , which constitutes clear orthologs of drosomycins. The multigene family encodes protein precursors of ~64 amino-acids with a signal peptide and mature peptides of 40–42 amino acids in their active form. Synthetic cremysin-5 exhibits therapeutic potential against human pathogenic yeasts. Further phylogenetic distribution analyses indicate that DTAFPs are not only present in Drosophila but are widely distributed to a clade of moulting animals (Ecdysozoa) [17] , including Arthropoda (Insecta, Entognatha, Myriapoda and Arachnida), Nematoda (Rhabditida and Tylenchida) and Tardigrada. These data allow for a more refined analysis of the origin and evolution of this class of disease resistance gene in animals. The discovery of new DTAFPs in nematodes To find whether there exist DTAFPs in non- Drosophila animals, we firstly searched the genomic BLAST databases of the Phylum Arthropoda in GenBank [14] by TBLASTN using drosomycins and plant defensins as queries. The databases include 63 species classified into four Classes (Insecta, Crustacea, Myriapoda and Arachnida) with 10 completely sequenced genomes, all derived from Insecta ( Supplementary Note 1 ). Consequently, we found that no species outside of the melanogaster species group of Drosophila contains DTAFPs, consistent with the previous observation [10] . On the basis of the Ecdysozoa hypothesis that nematodes are protostomes closely related to Drosophila and other arthropods [17] , our search scale thus extended to all the nematode genomic databases that include 20 species with two ( Caenorhabditis elegans and Caenorhabditis briggsae ) completely sequenced. The survey identified two species, the fruit nematode C. remanei and the Northern root-knot nematode Meloidogyne hapla , whose genomes contain genes encoding DTAFPs ( Fig. 1 ). 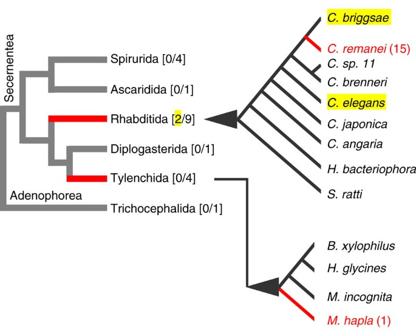Figure 1: Genomic BLAST searches identifying new DTAFPs in nematodes. The phylogenetic relationship of six nematode Orders from two Classes (Secernentea and Adenophorea), emphasizing Rhabditida and Tylenchida45. Species containing DTAFPs are shown in red and species with their genomes completely sequenced are shadowed in yellow. Species and gene numbers are indicated in square and round brackets, respectively, in which numbers of species with completely sequenced genomes are shadowed in yellow. Figure 1: Genomic BLAST searches identifying new DTAFPs in nematodes. The phylogenetic relationship of six nematode Orders from two Classes (Secernentea and Adenophorea), emphasizing Rhabditida and Tylenchida [45] . Species containing DTAFPs are shown in red and species with their genomes completely sequenced are shadowed in yellow. Species and gene numbers are indicated in square and round brackets, respectively, in which numbers of species with completely sequenced genomes are shadowed in yellow. Full size image Nematode DTAFPs are closely related to drosomycins From the draft genome of C. remanei strain PB4641, we identified a multigene family of DTAFPs comprising 15 members (herein termed cremycin-1 to cremycin-15) ( Fig. 2a ), in which 13 are tandem located on contig 182 within a region of~10 kb and two on contig 219.8 ( Fig. 2b ). All cremycin genes have a conserved gene structure composed of two exons and one intron of phase-1 that disrupts a positionally conserved amino-acid site located in the N-terminal loop ( Fig. 2a ; Supplementary Table 1 ). Cremycins share identical precursor organization with that of drosomycins and most plant defensins [3] , [11] , which is composed of an N-terminal hydrophobic signal peptide and a C-terminal mature peptide. All the mature peptides contain six conserved cysteines involved in three disulphide bridges. In comparison with most drosomycins and plant defensins, cremycins lack the fourth disulphide bridge, as in the case of several newly discovered orthologs of drosomycins in Drosophila takahashii ( Fig. 2a ). Cremycin-1 to cremycin-14 display high sequence similarity to each other but they have low similarity to cremycin-15 that has a unique amidated C-terminus due to the presence of a Gly-Arg motif [18] ( Fig. 2a ). 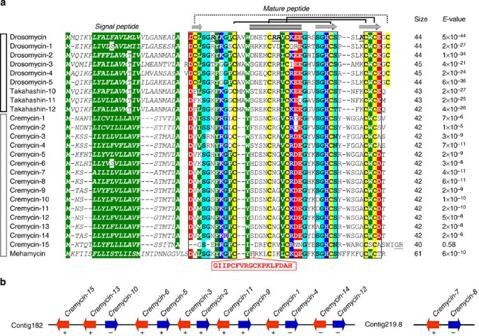Figure 2: DTAFPs in nematodes. (a) Multiple sequence alignment (MSA) showing evolutionary conservation of the precursor amino-acid sequences between nematode andDrosophila DTAFPs, where hydrophobic or aromatic amino acids are shadowed in green, hydrophilic residues in cyan, acidic residues and their conservative replacements in red, basic in blue and cysteines in yellow. Residues split by a positionally conserved phase-1 intron among nematode DTAFPs are boxed in pink. Four conserved blocks across the alignment are boxed in grey. Secondary structure elements (cylinder: α-helix; arrow: β-strand) and disulphide bridge connectivities are extracted from the structural coordinates of drosomycin (pdb entry 1MNY). The dotted line represents the disulphide bridge absent in some members. Functional sites of drosomycin are italicized and underlined once. DTAFPs fromDrosophila(D. melanogasterandD. takahashii) and nematodes (C. remaneiandM. hapla) are indicated by black and grey bars to the left of the alignment, respectively. A proposed insertion in mehamycin is boxed in red; (b) the arrangement ofcremycingenes in the chromosome ofC. remanei. Arrows in different colours refer to the orientation of the genes and the sign,+ or −, indicates transcription or no transcription when identified by RT–PCR (Fig. 4a). Figure 2: DTAFPs in nematodes. ( a ) Multiple sequence alignment (MSA) showing evolutionary conservation of the precursor amino-acid sequences between nematode and Drosophil a DTAFPs, where hydrophobic or aromatic amino acids are shadowed in green, hydrophilic residues in cyan, acidic residues and their conservative replacements in red, basic in blue and cysteines in yellow. Residues split by a positionally conserved phase-1 intron among nematode DTAFPs are boxed in pink. Four conserved blocks across the alignment are boxed in grey. Secondary structure elements (cylinder: α-helix; arrow: β-strand) and disulphide bridge connectivities are extracted from the structural coordinates of drosomycin (pdb entry 1MNY). The dotted line represents the disulphide bridge absent in some members. Functional sites of drosomycin are italicized and underlined once. DTAFPs from Drosophila ( D. melanogaster and D. takahashii ) and nematodes ( C. remanei and M. hapla ) are indicated by black and grey bars to the left of the alignment, respectively. A proposed insertion in mehamycin is boxed in red; ( b ) the arrangement of cremycin genes in the chromosome of C. remanei . Arrows in different colours refer to the orientation of the genes and the sign,+ or −, indicates transcription or no transcription when identified by RT–PCR ( Fig. 4a ). Full size image Sequence similarities among DTAFPs from C. remanei , Drosophila and plants are statistically highly significant with expectation values ( E -values) ranging from 3 × 10 −4 to 4 × 10 −11 ( Fig. 3a ). The level of significance of the E -values indicates that all these molecules are evolutionarily related. Clearly, cremycins are more closely related to drosomycins than to plant defensins according to their E -values ( Fig. 3a ), which is further supported by phylogenetic analysis of a total of 176 DTAFPs from C. remanei , Drosophila and plants ( Supplementary Data 1 ). In the trees constructed by the neighbour-joining (NJ) and maximum likelihood (ML) methods, crymycins and drosomycins cluster together with high bootstrap support ( Fig. 3b ), in line with sequence analyses by WebLogo [19] that identified 25 conserved sites between cremycins and drosomycins but only 18 such sites between cremycins and plant defensins ( Fig. 3c ). 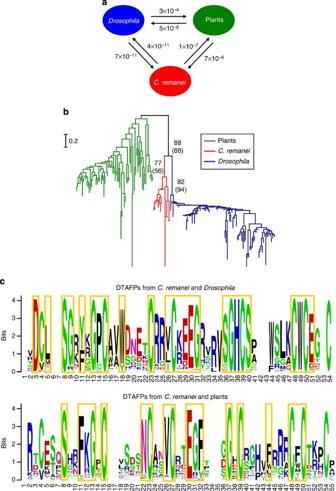Figure 3: Evolutionary relationship among DTAFPs from different origins. (a) Values correspond to BLASTE-values between DTAFPs from different origins. Arrows indicate the search direction; (b) the NJ tree resolving the relationship of DTAFPs. The scale bar indicates 0.2 substitutions per site. The topology of the tree is further confirmed by ML analysis with high bootstrap values (500 replicates) indicated in parentheses; (c) the sequence logo of DTAFPs, analysed by WebLogo19, identifying conserved sites (boxed in golden) betweenC. remaneiandDrosophilaor plants. Figure 3: Evolutionary relationship among DTAFPs from different origins. ( a ) Values correspond to BLAST E -values between DTAFPs from different origins. Arrows indicate the search direction; ( b ) the NJ tree resolving the relationship of DTAFPs. The scale bar indicates 0.2 substitutions per site. The topology of the tree is further confirmed by ML analysis with high bootstrap values (500 replicates) indicated in parentheses; ( c ) the sequence logo of DTAFPs, analysed by WebLogo [19] , identifying conserved sites (boxed in golden) between C. remanei and Drosophila or plants. Full size image Besides cremycins, we also identified a new DTAFP gene from the draft genome of M. hapla , a nematode species that diverged >500 million years ago (MYA) from Caenorhabditis [20] . This gene, named mehamycin , codes for a precursor with high sequence similarity to drosomycins and cremycins ( E -values from 1 × 10 −6 to 2 × 10 −9 ), indicating their evolutionary relationship, which is further supported by the conserved exon–intron structure between mehamycin and cremycins ( Fig. 2a ). Interestingly, the mature peptide of mehamycin is larger in size than that of these two classes of DTAFPs, as identified by an insertion of 18 amino acids between Cys1 and Cys2 ( Fig. 2a ). Functional features of nematode DTAFPs Reverse transcription PCR (RT–PCR) confirmed that 10 of 15 cremycin genes were transcriptionally active, in which four ( cremycin-5 , -9 , -11 and -15 ) were transcribed only after challenged by the fungus Neurospora crassa ( Fig. 4a ). In the absence of the fungus, cremycin-3 and -6 can also be transcribed, but their transcription level was upregulated after challenge. These observations indicate that the six genes are inducible by fungi. By contrast, cremycin-7 and -13 are two constitutive genes whose expression was not affected by the challenge ( Fig. 4a ; Supplementary Fig. 1 ). In our semiquantitative RT–PCR assay, cremycin-1 and -2 co-existed in the same PCR product due to their nearly identical sequences. Similar to cremycin-7 and -13 , cremycin-1 and -2 are also two constitutively expressed genes ( Fig. 4a ). Of the eight functional residues of drosomycin implicated in the interaction with fungi, seven previously identified [7] and one identified here ( Fig. 2a ; Supplementary Fig. 2 ), at least one-half are conserved in cremycin-1 to cremycin-14 ( Fig. 4b ) and only cremycin-15 exhibits more sequence divergence in the functional sites ( Fig. 2a ). 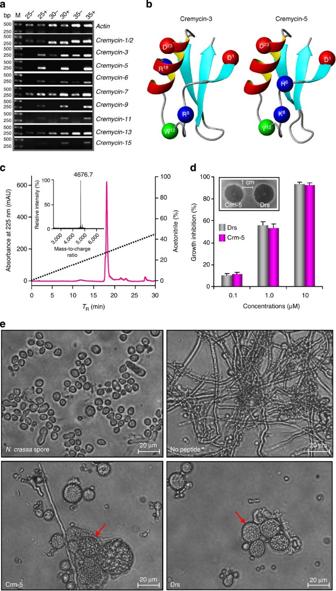Figure 4: Functional features of cremycins. (a) Cropped blots showing semiquantitative RT–PCR detection of the expression ofcremycingenes before and after fungal challenge. The complete blots are provided inSupplementary Fig. 1. Actin was used a control. All PCR products were amplified at an annealing temperature of 62 °C. M: DNA marker. −: non-challenged; +: challenged. Numbers represent PCR cycles; (b) ribbon diagrams of two cremycin structures modelled from drosomycin at the SWISS-MODEL server50. The Cαatoms of conserved residues corresponding to the functional sites of drosomycin are displayed using the Corey–Pauling–Koltun (CPK) representation; (c) reversed-phase high-pressure liquid chromatography (RP-HPLC) showing the retention time (TR) of chemically synthetic cremycin-5 in its oxidative form; matrix-assisted laser desorption ionization time-of-flight mass spectrometry (MALDI-TOF MS) shown in inset; (d,e) effects of cremycin-5 (Crm-5) and drosomycin (Drs) onN. crassa. (d) Concentration-dependent liquid growth inhibition. Data are expressed as mean±s.e. (n=3). Inhibition zones formed by 0.4 nmol of peptides each well are displayed in the inset. (e) Morphological damages ofN. crassaspores by 10 μM peptides. Photomicrographs were taken after 24 h of incubation of theN. crassaspore suspension in 1 × MEA in the absence or presence of the peptides. The damaged spores are indicated by red arrows. Figure 4: Functional features of cremycins. ( a ) Cropped blots showing semiquantitative RT–PCR detection of the expression of cremycin genes before and after fungal challenge. The complete blots are provided in Supplementary Fig. 1 . Actin was used a control. All PCR products were amplified at an annealing temperature of 62 °C. M: DNA marker. −: non-challenged; +: challenged. Numbers represent PCR cycles; ( b ) ribbon diagrams of two cremycin structures modelled from drosomycin at the SWISS-MODEL server [50] . The C α atoms of conserved residues corresponding to the functional sites of drosomycin are displayed using the Corey–Pauling–Koltun (CPK) representation; ( c ) reversed-phase high-pressure liquid chromatography (RP-HPLC) showing the retention time ( T R ) of chemically synthetic cremycin-5 in its oxidative form; matrix-assisted laser desorption ionization time-of-flight mass spectrometry (MALDI-TOF MS) shown in inset; ( d , e ) effects of cremycin-5 (Crm-5) and drosomycin (Drs) on N. crassa . ( d ) Concentration-dependent liquid growth inhibition. Data are expressed as mean±s.e. ( n =3). Inhibition zones formed by 0.4 nmol of peptides each well are displayed in the inset. ( e ) Morphological damages of N. crassa spores by 10 μM peptides. Photomicrographs were taken after 24 h of incubation of the N. crassa spore suspension in 1 × MEA in the absence or presence of the peptides. The damaged spores are indicated by red arrows. Full size image Cremycin-5 was selected for further functional characterization not only because it is a fungus-inducible gene but also because there was no precedent for a nematode DTAFP reported. In view of the more sequence divergence occurring between cremycin-15 and other paralogs, we also chose this peptide for a comparative study. We chemically synthesized these two peptides with a purity of more than 95%, as identified by reversed-phase high-pressure liquid chromatography and MALDI-TOF MS (matrix-assisted laser desorption ionization time-of-flight mass spectrometry) ( Fig. 4c ; Supplementary Fig. 3 ). Antimicrobial assays showed that cremycin-5 and drosomycin had similar potency against the filamentous fungus N. crassa ( Fig. 4d ) with a lethal concentrations ( C L ) of 0.3–0.6 μM ( Table 1 ) and a peptide concentration at half-maximal inhibition efficacy (IC 50 ) of 0.74–0.88 μM. At a higher concentration (10 μM) cremycin-5 damaged spores of N. crassa and inhibited their germination into hyphae ( Fig. 4e ), a typical effect previously observed in drosomycin [5] . Cremycin-5 was also active on other filamentous fungi: Geotrichum candidum ( C L : 4.7 μM), Aspergillus niger ( C L : 14.9 μM), three A. nidulans stains ( C L : 0.7–1.7 μM) ( Table 1 ). Remarkably, although cremycin-5 had a similar potency to drosomycin and drosomycin-2 against the yeast Saccharomyces cerevisiae ( C L : 5.5–8.9 μM), it exhibited more activity against two pathogenic yeasts ( Candida albicans and Candida tropicalis ) ( Table 1 ). This peptide was capable of inhibiting the growth of an array of clinical isolates of these two species ( C L : 1.8–26.0 μM). The effect of cremycin-5 on the viability of C. albicans 4287 was examined by an MTT (3-(4,5-Dimethylthiazol-2-yl)-2,5-Diphenyltetrazolium Bromide)-based cytotoxicity assay that measures the mitochondrial dehydrogenase activities of live cells in the formation of MTT/formazan crystals. After treatment with 5 × C L peptide, only 50% of the cells remained viable ( Fig. 5a ), indicating that the peptide is of fungicidal activity through a non-membrane disruption modes of action, as shown in Fig. 5b . Table 1 Comparison of lethal concentrations of nematode and Drosophila DTAFPs on different fungi. 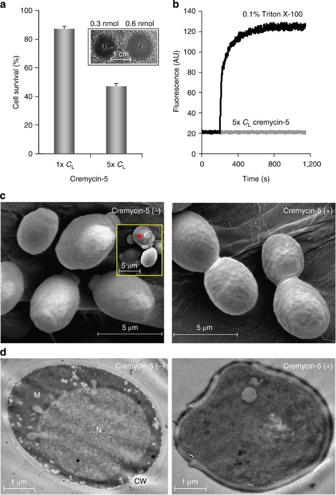Figure 5: Effects of cremycin-5 onC. albicans4287. (a) Cell viability ofC. albicansafter treatment with cremycin-5, monitored using an MTT-based assay. Data are expressed as mean±s.e. (n=3). Inhibition zones are shown in the inset; (b) effect of cremycin-5 on membrane integrity ofC. albicans. Triton X-100 was used as a positive control; (c) scanning electron micrographs ofC. albicanscells in the presence and absence of cremycin-5. The red arrow indicates budding of a normal cell; (d) transmission electron microscopic observation of effects of cremycin-5 onC. albicanscells. CW, cell wall; M, mitochondrion; N, nucleus. Full size table Figure 5: Effects of cremycin-5 on C. albicans 4287. ( a ) Cell viability of C. albicans after treatment with cremycin-5, monitored using an MTT-based assay. Data are expressed as mean±s.e. ( n =3). Inhibition zones are shown in the inset; ( b ) effect of cremycin-5 on membrane integrity of C. albicans . Triton X-100 was used as a positive control; ( c ) scanning electron micrographs of C. albicans cells in the presence and absence of cremycin-5. The red arrow indicates budding of a normal cell; ( d ) transmission electron microscopic observation of effects of cremycin-5 on C. albicans cells. CW, cell wall; M, mitochondrion; N, nucleus. Full size image Initial light microscopic observation suggested that cremycin-5 inhibited cytokinesis of C. albicans cells ( Supplementary Fig. 4 ). This is further verified by the scanning electron microscopic observation, in which treated cells were not capable of dividing into two single daughter cells due to the cytokinesis inhibited and the cells displayed rough surface. On the contrary, normal C. albicans cells without the peptide lie apart and each has one to several bud scars and smooth surface ( Fig. 5c ). Transmission electron microscopy (TEM) showed evident damages of cellular surfaces and intracellular structure of the treated cells ( Fig. 5d ). Similar to drosomycins, cremycin-5 is also a strict antifungal peptide without activity on bacteria used here at 50 μM. This peptide was able to retain activity after 24 h of incubation with 100% mouse serum and had no haemolysis even at 50 μM ( Supplementary Fig. 5 ). In contrast to cremycin-5, cremycin-15 inhibited the growth of two Gram-positive bacteria ( Bacillus megaterium and Serratia marcescens ) at C L of 14.1–17.7 μΜ, but it exhibited no activity on the fungi used here ( Supplementary Table 2 ), implying functional diversification between paralogous cremycins after gene duplication. Despite the presence of a small insertion relative to cremycins and drosomycins, mehamycin appears to be also a functional gene because it has been confirmed to be transcriptionally active in the expressed sequence tag (EST) database (CF370770), and among the eight functional residues of drosomycin, six are conserved or conservative replacements in mehamycin ( Fig. 2a ). Restricted distribution of DTAFPs in ecdysozoans It has been previously shown that there are drosomycin-like sequences from non- Drosophila insects in the EST database, which were isolated from complementary DNA (cDNA) libraries of three coleopteran species ( Callosobruchus maculates , Trox sp. JH-2005 and Agriotes lineatus ) [10] . To rule out potential contamination, we used C. maculates as an example to amplify its genomic DNA. As a result, we identified two positive clones, one coding for a DTAFP precursor with identical amino-acid sequence to that depicted in the EST database ( C. maculates -1) and another coding for a new DTAFP with several point mutations ( C. maculates -3) ( Fig. 6a ). In addition, our BLASTP search retrieved a hit from Musca domestica that has identical sequence to drosomycin. We also confirmed its presence in the M. domestica genome by PCR amplification and DNA sequencing ( Fig. 6b ). 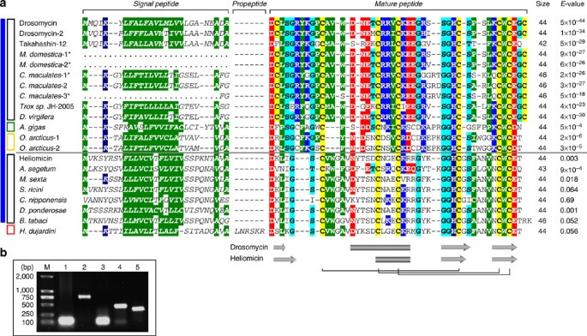Figure 6: New DTAFPs from non-DrosophilaArthropoda and Tardigrada. (a) MSA highlighting the conservation of amino-acid sequences. Colour codes are detailed inFig. 2a. Secondary structure elements and disulphide bridge connectivities are extracted from structural coordinates of drosomycin and heliomicin (pdb entry 1I2U). The drosomycin and heliomicin families are distinguished by a grey line. DTAFPs from different origins are indicated by bars in colour (black: Insecta; green: Myriapoda; gold: Entognatha; red: Tardigrada; blue: Arthropoda) to the left of the alignment. ‘...’ represents undetermined sequences. With the exception ofM. domestica-1,M. domestica-2,C. maculates-3 (Supplementary Fig. 6) andC. maculates-1 (KF429250) which all are cloned in this work (indicated by ‘*’), other non-Drosophilapeptides all are retrieved from GenBank14:C. maculates-2 (FK669231),Troxsp. JH-2005 (DV767586),D. virgifera virgifera(EW769059),A. gigas(FN197359),O. arcticus-1 (EW757012),O. arcticus-2 (EW758773), heliomicin (GT206445),A. segetum(ES584181),M. sexta(ADQ00386),S. ricini(DC870370),S. ricini(DC870370),C. nipponensis(FE527725),D. ponderosae(GT484290),B. tabaci(AGE89239), andH. dujardini(CK326749). The sequence ofA. lineatus(CV160723) is not included here due to its incomplete mature peptide; (b) genomic amplification ofdrosomycininD. melanogaster,M. domesticaandC. maculates. M, DNA marker; Lane 1:D. melanogastergDNA — drosomycin; 2:M. domesticagDNA — 28 S rDNA; 3:M. domesticagDNA — drosomycin; 4:C. maculatesgDNA — 28 s rDNA; 5:C. maculatesgDNA — drosomycin. Figure 6: New DTAFPs from non- Drosophila Arthropoda and Tardigrada. ( a ) MSA highlighting the conservation of amino-acid sequences. Colour codes are detailed in Fig. 2a . Secondary structure elements and disulphide bridge connectivities are extracted from structural coordinates of drosomycin and heliomicin (pdb entry 1I2U). The drosomycin and heliomicin families are distinguished by a grey line. DTAFPs from different origins are indicated by bars in colour (black: Insecta; green: Myriapoda; gold: Entognatha; red: Tardigrada; blue: Arthropoda) to the left of the alignment. ‘...’ represents undetermined sequences. With the exception of M. domestica -1, M. domestica -2, C. maculates -3 ( Supplementary Fig. 6 ) and C. maculates -1 (KF429250) which all are cloned in this work (indicated by ‘*’), other non- Drosophila peptides all are retrieved from GenBank [14] : C. maculates -2 (FK669231), Trox sp. JH-2005 (DV767586), D. virgifera virgifera (EW769059), A. gigas (FN197359), O. arcticus -1 (EW757012), O. arcticus -2 (EW758773), heliomicin (GT206445), A. segetum (ES584181), M. sexta (ADQ00386), S. ricini (DC870370), S. ricini (DC870370), C. nipponensis (FE527725), D. ponderosae (GT484290), B. tabaci (AGE89239), and H. dujardini (CK326749). The sequence of A. lineatus (CV160723) is not included here due to its incomplete mature peptide; ( b ) genomic amplification of drosomycin in D. melanogaster , M. domestica and C. maculates . M, DNA marker; Lane 1: D. melanogaster gDNA — drosomycin; 2: M. domestica gDNA — 28 S rDNA; 3: M. domestica gDNA — drosomycin; 4: C. maculates gDNA — 28 s rDNA; 5: C. maculates gDNA — drosomycin. Full size image On the basis of the discovery of DTAFPs outside of Drosophila , we further carried out TBLASTN screen of the EST database by using drosomycins and cremycins as queries, which yielded significant hits from several non- Drosophila species. One sequence from the giant African millipede Archispirostreptus gigas (Myriapoda) exhibits E -values of 5 × 10 −4 to drosomycins and 7 × 10 −5 to cremycins, whereas two sequences from the Arctic springtail Onychiurus arcticus (Entognatha) exhibit E -values of 2 × 10 −6 to drosomycins and 9 × 10 −13 to cremycins. This new cycle of search also identified another DTAFP from the coleopteran Diabrotica virgifera virgifera ( Fig. 6a ). In addition to the hits described above with significant E -values, some hits with low sequence similarity ( E -values of 2.6–9 × 10 −4 ) should also be considered as remote homologues of DTAFPs due to the similarity in structure and function, according to the criteria of Russell et al. [21] All these hits are heliomicin-like antifungal peptides with a CSαβ-fold [22] . Their evolutionary relationship with DTAFPs is strengthened by the discovery that heliomicin and plant defensins interact with the same target in the fungal plasma membrane [23] . These newly discovered sequences are distributed in four Orders of Insecta (Arthopoda) that include Lepidoptera, Hemiptera, Neuroptera and Coleoptera, and species from Tardigrada ( Fig. 6a ). Functional diversification of DTAFPs in the scorpion lineage Our BLAST search also retrieved several scorpion toxins with similar sequences to drosomycins ( E -values from 1 × 10 −3 to 4 × 10 −6 ). These molecules belong to a family of scorpion toxins affecting sodium channels ( Fig. 7a ). They have an unusual structure that is composed of a conserved core folding into a drosomycin-like scaffold and an NC-domain comprising the N-terminal turn (N-turn) and C-tail [24] ( Fig. 7b ). Experimental deletion of the NC-domain of a scorpion toxin resulted in antifungal ability of the toxin [25] , whereas the addition of the NC-domain of a toxin on the drosomycin scaffold led to a neurotoxin targeting rat sodium channels [26] . These data provide convincing functional evidence in favour of evolutionary link between drosomycins and scorpion sodium channel toxins, and present an example of divergent evolution occurring in a specific arthropod lineage, in which a DTAFP evolved into a neurotoxin [24] , [25] , [26] . The insertion of a small fragment, as the N-turn of the scorpion toxins, in the N-terminal region of a DTAFP is also seen in mehamycin ( Fig. 2a ) despite its function remains to be characterized. 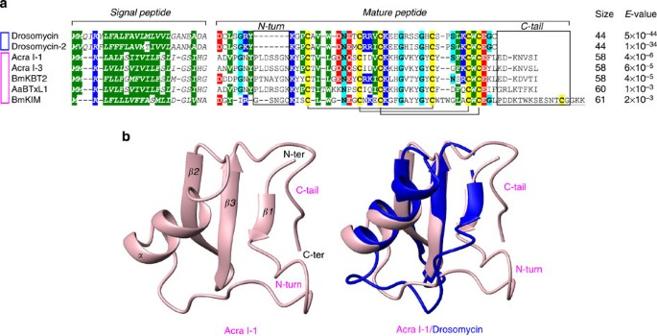Figure 7: Scorpion sodium channel toxin-like peptides are closely related to drosomycins. (a) MSA highlighting the conservation of amino-acid sequences. Colour codes are detailed inFig. 2a. N-turn and C-tail specific in scorpion toxins are boxed; (b) structural superimposition of drosomycin and AcraI-1, a toxin from the scorpionAndroctonus crassicauda, highlighting the toxin-specific regions (N-ter and C-ter). The model of AcraI-1 was built from the structure of Cn5 (pdb entry 2KJA), a crustacean toxin found in the venom of the scorpionsC. noxiusandC. suffusus suffuses51. The GenBank accession numbers of toxin sequences are AcraI-1 (P0C293), AcraI-3 (P0C294), BmKBT2 (AF151798), AaBTxL1 (Q4LCS8) and BmKIM (Q8I0K7). Figure 7: Scorpion sodium channel toxin-like peptides are closely related to drosomycins. ( a ) MSA highlighting the conservation of amino-acid sequences. Colour codes are detailed in Fig. 2a . N-turn and C-tail specific in scorpion toxins are boxed; ( b ) structural superimposition of drosomycin and AcraI-1, a toxin from the scorpion Androctonus crassicauda , highlighting the toxin-specific regions (N-ter and C-ter). The model of AcraI-1 was built from the structure of Cn5 (pdb entry 2KJA), a crustacean toxin found in the venom of the scorpions C. noxius and C. suffusus suffuses [51] . The GenBank accession numbers of toxin sequences are AcraI-1 (P0C293), AcraI-3 (P0C294), BmKBT2 (AF151798), AaBTxL1 (Q4LCS8) and BmKIM (Q8I0K7). Full size image In this study, we report the discovery of a multigene family of DTAFPs in a fruit nematode based on evolutionary genomics and experimental approaches. To our knowledge, this is the first report that describes functional DTAFPs in a non- Drosophila animal. The activity of cremycin-5 against a series of clinical isolates of the human pathogens ( C. albicans and C. tropicalis ), together with high serum stability and no haemolysis, makes it a promising therapeutic drug lead. A combination of molecular cloning and exhaustive database searches revealed that animal DTAFPs actually have a wider phylogenetic distribution than initially thought. The most interesting finding in this work is that all species identified here possessing DTAFPs belong to the Ecdysozoa, a clade of moulting animals, which includes three phyla (Arthropoda, Nematoda and Tardigrada) [17] , [27] . The restricted presence in Ecdysozoa together with the widespread distribution in plants and the absence in fungi and protozoans indicates a patch distribution pattern of this gene in eukaryotes ( Fig. 8 ). If such a pattern is a consequence of vertical heredity, this would require that the last common ancestor of all eukaryotes evolved this gene and then it lost independently in fungi and all metazoans except ecdysozoans after the divergence of the main eukaryotic lineages. In this case, one could predict that protozoans, the early-diverged eukaryotes and the supposed common ancestor of metazoans [28] , would contain DTAFPs. However, a detailed survey of all the sequenced protozoan genomes of 134 species (strains) including 22 species (strains) with completely sequenced genomes ( Supplementary Note 1 ) failed to find any significant hits. In the work of Roelofs and van Haastert [29] , the discovery of 11 genes shared by the protozoan Dictyostelium and human has been used as evidence to exclude HGT from bacteria to human and to support divergent evolution. The clear absence of this gene in protozoans implies that DTAFPs were not evolved in early animals. 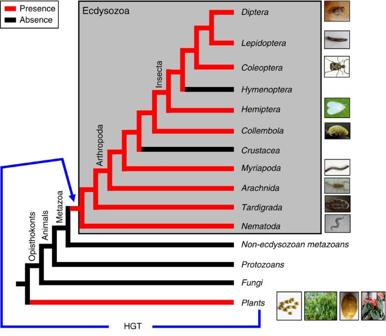Figure 8: Patch distribution and proposed HGT of DTAFPs. The tree of Eukaryotes is a summary of diverse sources, with emphasis on Ecdysozoa, in which branches containing species with DTAFPs are shown in red. HGT from plants to the common ancestry of Ecdysozoa is indicated by blue arrow. Photographs ofC. remaneiandC. maculatesare kindly provided by Dr Nadine Timmermeyer and Prof. Georg Goergen, respectively. Figure 8: Patch distribution and proposed HGT of DTAFPs. The tree of Eukaryotes is a summary of diverse sources, with emphasis on Ecdysozoa, in which branches containing species with DTAFPs are shown in red. HGT from plants to the common ancestry of Ecdysozoa is indicated by blue arrow. Photographs of C. remanei and C. maculates are kindly provided by Dr Nadine Timmermeyer and Prof. Georg Goergen, respectively. Full size image Because of a monophyletic origin of the Ecdysozoa [27] , we thus believe that one HGT from plants to ecdysozoans would be by far the most favoured explanation ( Fig. 8 ). This is highly coincided with their divergence times. It is estimated that higher plants diverged from chlorophytan green algae at 968±93 MYA [30] or 1061±109 MYA [31] and the fundamental split within higher plants occurred at the Cryogenian period (670 MYA) [32] , earlier than an Ediacaran origin of all major ecdysozoan lineages (~587–543 MYA) [33] . It is likely that the evolution of a DTAFP first in plants, which was then transferred to the common ancestor of Ecdysozoa and subsequently diversified into its constituent phyla. This is consistent with the phylogentic tree ( Fig. 3b ), where DTAFPs from nematodes and Drosophila form two separate clusters but they both are closer to each other than to plant defensins. It has been shown that the nematodes frequently gained new introns during evolution [34] . This is the case for cremycins and mehamycin ( Fig. 2a ). In contrary to drosomycins that lack an intron, nematode DTAFPs gained a conserved phase-1 intron before the divergence of C. remanei and M. hapla , supporting vertical evolution of this gene in nematodes. An ancient HGT followed by speciation and divergence is also observed in the aphid carotenoid synthetic genes that were presumably obtained from a fungus by HGT [35] . Despite this, the fact that the two nematode species with DTAFPs literally roll around decomposing plant matter in most of their reproductive lives suggests that the alternative possibility of two independent introductions of these defensive peptides to C. remanei and M. hapla by HGT from plants can be not completely ruled out. It is also worth mentioning that the patch distribution of DTAFPs among the distantly related species could result from evolutionary convergence for defence against fungi. If so, this would require that all these molecules are derived from independent genetic starting points, as in the case of a defensive peptide that has been evolved from two evolutionarily unrelated genes in two distantly related frog species [36] . However, high sequence, structural and functional similarity together with identical precursor organization (a signal peptide followed by a mature peptide) provides more support for their evolutionary relationship other than molecular convergence. To draw a decisive conclusion on evolutionary relationship or convergence, one could need more completely sequenced genomes of ecdysozoans to investigate the precise distribution of DTAFPs. Although present in plants and ecdysozoans, the evolution of DTAFPs appears to be more successful in plants than in ecdysozoans based on their differential phylogenetic distribution. From an ecological point of view, such evolutionary success could be due to the symbiosis of fungi and plants in natural ecosystems [37] providing a selective force to maintain retention of the antifungal gene during plant evolution. This is also true for some species of ecdysozoans, such as Drosophila and C. remanei , which both live in fungi-rich rotting fruits [1] , [16] and thus facilitates the retention of multiple DTAFP genes in their genomes. However, some other species of insects and nematodes have lost this gene, as evidenced by the absence of any orthologs in their completely sequenced genomes, such as Nasonia vitripennis , Apis mellifera , Bombus terrestris , Anopheles gambiae , Tribolium castaneum , C. elegans , and C. briggsae . The loss of DTAFPs in these species suggests its poor fixation during ecdysozoan evolution. This could be partly explained by the absence of selective pressure in several insects that live in a fungi-poor environment, such as N. vitripennis and A. gambiae . In fact, the lack of microbes in its niches has been considered as a cause leading to the loss of many antimicrobial genes during aphid evolution [38] . However, considering key immune roles of DTAFPs in resisting fungal infection [6] , [11] , the loss of this gene in two sibling species of C. remanei ( C. elegans and C. briggsae ) is puzzling as they also live in fungi-rich habitats. A potential explanation is that these two nematode species could mount an alternative, but equal, antifungal genes. In fact, microarray-based transcriptional profiling of infected worms combined with computational approaches has identified seven fungus-induced peptide ( fip ) genes and 29 fip -related genes in C. elegans [39] . Alternatively, differential fixation of DTAFPs in different species of Caenorhabditis could be a reflection of their diverse ecologies [40] . For example, despite C. elegans and C. briggsae both exist in large, proliferating populations in rotting fruits and stems, their temporal distributions do not coincide [41] . In addition, C. remanei and the two sibling species exhibit totally different reproduction modes. Different from the gonochoristic C. remanei , C. elegans and C. briggsae have evolved a self-fertile hermaphroditic mode. Because evolutionary transitions between sexual modes are potent forces in genome evolution [42] , this could be another cause for the differential fixation of the gene in these three species. The absence of DTAFPs in C. elegans and C. briggsae is consistent with the genome shrinkage in these two selfing species [42] . Extensive gene duplication to assemble a multigene family is a typical feature observed in many genes transferred to the nematode genomes [43] . In plants and the ecdysozoans with this gene, most of DTAFPs also exist as multigene families and some have evolved novel biological functions. For example, in addition to major antifungal activity, some plant DTAFPs have developed diverse activities as inhibitors of protein translation, enzymes and bacterial growth, mediators of zinc tolerance, and blockers of ion channels [44] . Similarly, drosomycin has been found to gain ability in interacting with the fly voltage-gated sodium channel, possibly acting as a neuropeptide [25] . In C. remanei , cremycin-15 has evolved antibacterial activity described here, while scorpion venom-derived DTAFPs have switched their targets from fungi to animal sodium channels [24] , [25] , [26] . All these observations suggest that the gene can be fixed only in organisms where it developed important functions following gene duplication and speciation. In conclusion, our work has revealed a complex evolutionary history of DTAFPs, in which an ancient HGT from plants led to the origin of a disease resistance gene in a specific animal clade and subsequent vertical inheritance involving gene duplication, loss and functional diversification shaped this gene family in ecdysozoans. Our discovery might be also valuable in guiding the discovery of new DTAFPs with therapeutic potential from other ecdysozoans living in fungi-rich niches. Database search To find new DTAFPs, we first used the amino-acid sequences of drosomycins and plant defensins as queries to perform TBLASTN search of the genomic BLAST databases in GenBank under default parameters [14] . The database contains 20 species of Nematoda with two genomes completely sequenced ( C. briggsae and C. elegans ) ( Supplementary Note 1 ). These species belong to five Orders of Class Secernentea (Ascaridida, Spirurida, Tylenchida, Rhabditida and Diplogasterida) and one Order of Class Adenophalida [45] (Trichocephalida). The database also contains 62 species of the Phylum Arthropoda with ten completely sequenced insect genomes ( Anopheles gambiae str. PEST, D. melanogaster , D. pseudoobscura pseudoobscura , D. simulans , D. yakuba , Tribolium castaneum , Apis mellifera , Bombus terrestris , Nasonia vitripennis , and Acyrthosiphon pisum ) ( Supplementary Note 1 ). Using the same approaches presented here, we also searched other databases in GenBank, which include the nucleotide collection (nr/nt) database, the EST database, and the reference genomic sequences (refseq_genomic) database [14] . The database E -values were calculated by the BLAST programs using the equation: E=N /2 S ′ , where N is the total length of the database in residues and S ′ is the normalized score for a high-scoring segment pair (HSP) [46] . Phylogenetic tree constructions Amino-acid sequences of DTAFPs from Drosophila , C. remanei and plants ( Supplementary Data 1 ) were aligned by ClustalX, which were then used to construct phylogenetic trees by the NJ and ML methods in MEGA 5.0 (ref. 47 ), on the basis of the Jones–Taylor–Thornton substitution model with a gamma distribution of rates between sites. In ML analysis, an initial tree was first built automatically with the NJ method and then variants of the topology were created with the nearest neighbour interchange method to search for topologies for fitting the data better. Five hundred bootstrap replicates were performed in the NJ and the ML tree. Gene cloning and semiquantitative RT–PCR The TRIZOL reagent (SBS Genetech, Beijing) was used to prepare total RNA of C. remanei strain PB4641 according to the supplier’s instructions. Reverse transcription of mRNAs into the first-strand cDNAs was performed using EasyScript First-Strand cDNA Synthesis Kit (TransGen Biotech., Beijing) that was used as template for PCR amplification. PCR products were ligated into the pGM-T Vector and recombinant plasmids were transformed into Escherichia coli DH5a. Positive clones were sequenced with T7 or SP6 primer. Nucleotide sequences of cremycin-1 , cremycin-2 , cremycin-3 , cremycin-5 , cremycin-6 , cremycin-7 , cremycin-9 , cremycin-11 , cremycin-13 , and cremycin-15 have been deposited in the GenBank database under the accession numbers JN230817–JN230826, respectively. For semiquantitative RT–PCR, a cremycin gene was amplified from non-challenged cDNAs of C. remanei strain PB4641 or N. crassa -challenged cDNAs by a gene-specific primer and 3AP. PCR products obtained from different cycles (25, 30 and 35) were taken for comparison of the amounts of these products. The C. remanei actin was chosen as an internal control that was amplified by primers CRM-actin/3AP and the same cDNA templates. Primers are provided in Supplementary Table 2 . Chemical synthesis and oxidative refolding Cremycin-5 and cremycin-15 were chemically synthesized in their reduced form by ChinaPeptides Co. Ltd. (Shanghai, China). For oxidative refolding, peptide samples were dissolved in 0.1 M Tris–HCl buffer (pH 8.5) to a final concentration of 1 mM and incubated at 25 °C for 48 h. Peptides were purified to homogeneity by reversed-phase high-pressure liquid chromatography using a C 18 column. The column was equilibrated with 0.1% trifluoroacetic acid and purified products were eluted from the column with a linear gradient from 0% to 60% acetonitrile in 0.1% trifluoroacetic acid within 40 min. Molecular mass of peptides were determined by MALDI-TOF MS on a Kratos PC Axima CFR plus (Shimadzu Co. LTD, Kyoto, Japan). Antimicrobial assays For inhibition zone assays, fungi were incubated on 1 × MEA (malt extract agar) plate at 28 °C for 1 week. Spores were harvested and suspended in sterile water with an OD 595 of 0.5. Six ml of 1 × MEA containing 0.8% agarose was mixed with 50 μl spores suspension and poured into one Petri dish of 9.0 cm in diameter. Wells with a diameter of 3 mm were punched into the medium, filled with 2 μl of sample each well. The plate was incubated in dark at 28 °C for 24 h. Similar procedures were also used in antibacterial assays, in which MEA was replaced by Luria Broth medium and the incubation temperature was 37 °C instead of 28 °C. C L of peptides was determined by the inhibition-zone assays and IC 50 was defined as peptide concentration leading to 50% of fungal growth inhibition [48] . The sources of the microorganisms used in this assay are listed in Supplementary Table 3 . Haemolytic effect and serum stability Haemolytic effects of peptides against fresh mouse erythrocytes were assayed according to the standard method [49] . To assess serum stability, peptides were incubated in water or fresh mouse serum for 0, 1, 3, 6 and 24 h at 28 °C. Residual activities on N. crassa were measured by the inhibition zone assays. MTT assay To determine the viability of C. albicans cells treated by cremycin-5, the cells were incubated with MTT for 4 h. Pellets collected by centrifugation were dissolved in 200 μl dimethyl sulfoxide, and cell viability was measured at 570 nm by the VersaMax reader (Molecular Devices). Membrane permeability assay To assess the permeation ability of cremycin-5 on C. albicans cells, 5 × 10 5 cells in 500 μl of phosphate-buffered saline (PBS) were mixed with propidium iodide to a final concentration of 1 μM for 5 min in the dark. After peptide was added, the absorbance was measured by a F-4500 fluorescence spectrophotometer (Hitachi High-Technology Company). Once basal fluorescence reached a constant value, cremycin-5 or Triton X-100 was added. Changes in fluorescence absorbance were monitored and plotted as arbitrary units. Electron microscopy C. albicans cells were treated with cremycin-5 at 5 × C L at 30 °C for 90 min and were then fixed with 2.5% glutaraldehyde for 1 h and washed three times with PBS. For scanning electron microscopy (SEM), cells were dehydrated with a series of graded ethanol solution and then dried by BAL-TEC CPD030 critical point dryer before being mounted on carbon tape, sputtered with platinum coating (BAL-TEC SCD005). Images were visualized in FEI QUANTA 200. For TEM, cells were postfixed with 1% osmium tetroxide for 1 h. After washed twice with PBS, cells were dehydrated with a series of graded ethanol solution and then embedded in EPON 812 resin. Ultrathin sections were obtained by Leica EM UC6 t FC6 and stained with uranyl acetate and lead citrate. Images were visualized in a Tecnai Spirit 120 KV microscope. Accession codes: Nucleotide sequences of cremycin-1 , cremycin-2 , cremycin-3 , cremycin-5 , cremycin-6 , cremycin-7 , cremycin-9 , cremycin-11 , cremycin-13 , and cremycin-15 have been deposited in the GenBank/EMBL/DDBJ nucleotide core database under accession codes JN230817 to JN230826 . How to cite this article: Zhu, S. and Gao, B. Nematode-derived drosomycin-type antifungal peptides provide evidence for plant-to-ecdysozoan horizontal transfer of a disease resistance gene. Nat. Commun. 5:3154 doi: 10.1038/ncomms4154 (2014).